Magneto-fluorescent core-shell supernanoparticles Magneto-fluorescent particles have been recognized as an emerging class of materials that exhibit great potential in advanced applications. However, synthesizing such magneto-fluorescent nanomaterials that simultaneously exhibit uniform and tunable sizes, high magnetic content loading, maximized fluorophore coverage at the surface and a versatile surface functionality has proven challenging. Here we report a simple approach for co-assembling magnetic nanoparticles with fluorescent quantum dots to form colloidal magneto-fluorescent supernanoparticles. Importantly, these supernanoparticles exhibit a superstructure consisting of a close-packed magnetic nanoparticle ‘core’, which is fully surrounded by a ‘shell’ of fluorescent quantum dots. A thin layer of silica coating provides high colloidal stability and biocompatibility, and a versatile surface functionality. We demonstrate that after surface pegylation, these silica-coated magneto-fluorescent supernanoparticles can be magnetically manipulated inside living cells while being optically tracked. Moreover, our silica-coated magneto-fluorescent supernanoparticles can also serve as an in vivo multi-photon and magnetic resonance dual-modal imaging probe. The design and fabrication of materials that simultaneously contain more than one functional component, so-called multifunctional materials, is an active research area with the potential to have an impact on a wide range of technological applications [1] , [2] , [3] , [4] . Among a variety of possible building blocks, colloidal nanocrystals have proven to be ideal for generating higher-order architectures either in random or ordered assemblies [5] , [6] , [7] , [8] , [9] , [10] , [11] , [12] . In particular, co-assembling two types of nanocrystals with distinct properties into larger colloidal particles, especially at the mesoscopic scale, offers the possibility of producing new classes of nanoparticles (that is, supernanoparticles (SPs)) with a set of combined properties, all the while maintaining the colloidal nature of their building blocks [13] . Moreover, synthesizing SPs with well-defined internal structures, although challenging, may be critical in generating novel properties. In particular, magneto-fluorescent particles have been recognized as an emerging class of materials that have potential in advanced applications [3] , [14] , [15] , [16] , [17] . To fully realize their potential and to optimize their performance, the following design criteria need to be simultaneously fulfilled: uniform and tunable sizes, high magnetic content loading for synergistic magnetic properties, maximized loading of fluorophores at the surface for an optimized fluorescence signal, long-term colloidal stability and a versatile surface functionality for the varied requirements of different applications, especially in biology. A simple and versatile synthetic strategy gives the additional benefit of a relatively rapid materials fabrication. In the past decade, much effort has been devoted to developing synthetic strategies for the fabrication of such magneto-fluorescent materials, including heterostructure crystal growth [18] , [19] , [20] , [21] , co-encapsulation into organic structures (for example, oil droplet, lipid micelle and block co-polymer) or inorganic materials (for example, silica) [22] , [23] , [24] , [25] , [26] , [27] , [28] , [29] , template-based synthesis via either chemical bonding or physical attachment [30] , [31] , [32] . Our method is based on co-assembling CdSe-CdS core-shell quantum dots (QDs) with Fe 3 O 4 magnetic nanoparticles (MNPs) into colloidal SPs. In this co-assembly process, close-packed MNPs form a ‘core’ that is subsequently coated with a ‘shell’ of QDs, resulting in the formation of ‘core-shell’ structured SPs (CS-SPs). Additional thermal treatment transforms the randomly assembled ‘core’ MNPs into a periodic assembly with a face-centred-cubic (fcc) superlattice. The CS-SPs can be overcoated with a thin silica layer, offering them further surface functionality and colloidal stability. Importantly, these silica-coated CS-SPs (silica-CS-SPs) exhibit uniform and tunable sizes, high magnetic content loading, maximized fluorophore loading on the surface, substantial colloidal stability and versatile surface functionality. We demonstrate that after functionalizing with polyethylene glycol (PEG), silica-CS-SPs can be magnetically manipulated inside living cells while being optically tracked. Moreover, our silica-CS-SPs can also serve as a dual-modal imaging probe for in vivo multi-photon (MP) and magnetic resonance (MR) imaging. CdSe-CdS core-shell QDs (9.0±0.4 nm) and superparamagnetic Fe 3 O 4 MNPs (5.9±0.3 nm) were used to demonstrate the formation of multifunctional magneto-fluorescent SPs ( Supplementary Fig. 1 ). As shown schematically in Fig. 1a , hydrophobic QDs and MNPs were mixed and transferred to an aqueous solution using dodecyltrimethylammonium bromide (DTAB) as a surfactant. The resultant micelle aqueous solution was quickly injected into a poly(vinylpyrrolidone) (PVP) ethylene glycol (EG) solution. After 30 min of stirring, the PVP-stabilized SPs were isolated by centrifugation and re-dispersed into ethanol. Large-area transmission electron microscopy (TEM) and scanning electron microscopy (SEM) images show that the resulting spherical SPs have an average diameter of ~120 nm ( σ ~11%) ( Fig. 1b and Supplementary Fig. 2 ). Dynamic light scattering measurements give a hydrodynamic (HD) diameter of ~170 nm for ethanol-dispersed SPs ( Supplementary Fig. 3 ). The apparent increased HD diameter relative to that in TEM and SEM is due to the presence of a PVP polymer surface layer and its low contrast in TEM and SEM imaging. Higher magnification TEM images demonstrate that each SP is composed of close-packed nanoparticles ( Fig. 1c ). Owing to the uniformity of the QD and MNP building blocks ( σ ~4.4% for QDs and σ ~5.0% for MNPs) and their different sizes (9.0 nm for QDs and 5.9 nm for MNPs) ( Supplementary Fig. 1 ), the QDs and MNPs can be easily distinguished in TEM. TEM images in Fig. 1c,d illustrate that each SP contains both QDs and MNPs. This result is consistent with a series of additional observations including absorption and photoluminescence (PL spectra ( Fig. 1e ), wide angle X-ray diffraction ( Fig. 1f ), particle movement under external magnetic attraction ( Fig. 1g ) and energy dispersive X-ray spectroscopy ( Fig. 1h ). Energy dispersive X-ray spectroscopy gives an elemental composition of 27.3% cadmium and 72.7% iron, in agreement with the initially introduced quantities of QDs and MNPs ( Fig. 1h , inset). A phase separation occurs inside each SP, in which MNPs preferentially assemble to form a magnetic ‘core’, with the QDs forming a fluorescent ‘shell’ ( Fig. 1c,d ). Scanning TEM elemental mapping and line scan ( Fig. 1i,j ), and high-resolution TEM characterization ( Supplementary Fig. 4 ) further demonstrate this ‘core-shell’ superstructure. Three-dimensional TEM tomography is also consistent with only MNPs inside the SP core ( Supplementary Movie 1 ). With these observations, we speculate that the formation of this super ‘core-shell’ structure is most probably driven by enhanced forces, which originate from the magnetic dipole–dipole interactions of MNPs (that is, Fe 3 O 4 MNPs) in addition to the solvophobic interactions that drive the assembly of both MNPs and QDs ( Fig. 1a ). The same protocol, but with small QDs (6.0±0.3 nm) and large MNPs (9.6±0.4 nm), yields the same CS-SP architecture (small QDs as ‘shell’ and large MNPs as ‘core’) ( Supplementary Fig. 5 and Supplementary Movie 2 ). This control experiment excludes particle size as the dominant parameter for the formation of the ‘core-shell’ superstructure. 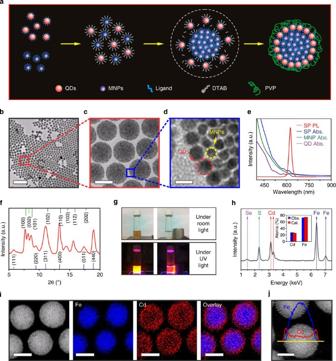Figure 1: Synthesis and characterizations of core-shell-structured SPs. (a) Schematic of the formation of the CS-SPs. (b–d) A set of TEM images of CS-SPs at different magnifications. Scale bars, 500 nm, 100 nm and 10 nm (b–d), respectively. (e) Absorption spectra of CS-SPs (blue), MNPs (green), QDs (purple) and photoluminescence spectrum of CS-SPs (red). (f) Wide-angle X-ray scattering pattern of CS-SPs. The stick patterns show the standard peak positions of bulk Fe3O4(magnetite, bottom blue sticks) and wurtzite CdS (top green sticks). (g) Photographs demonstrating the magnetic attraction of CS-SPs in the presence of a magnet under both room and ultraviolet light. (h) EDS spectrum of CS-SPs shown inb–d. (i) Images of dark-field scanning TEM and EDS elemental mapping from CS-SPs. Scale bars, 80 nm. (j) EDS elemental line scan result. Scale bar, 60 nm. Figure 1: Synthesis and characterizations of core-shell-structured SPs. ( a ) Schematic of the formation of the CS-SPs. ( b – d ) A set of TEM images of CS-SPs at different magnifications. Scale bars, 500 nm, 100 nm and 10 nm ( b – d ), respectively. ( e ) Absorption spectra of CS-SPs (blue), MNPs (green), QDs (purple) and photoluminescence spectrum of CS-SPs (red). ( f ) Wide-angle X-ray scattering pattern of CS-SPs. The stick patterns show the standard peak positions of bulk Fe 3 O 4 (magnetite, bottom blue sticks) and wurtzite CdS (top green sticks). ( g ) Photographs demonstrating the magnetic attraction of CS-SPs in the presence of a magnet under both room and ultraviolet light. ( h ) EDS spectrum of CS-SPs shown in b – d . ( i ) Images of dark-field scanning TEM and EDS elemental mapping from CS-SPs. Scale bars, 80 nm. ( j ) EDS elemental line scan result. Scale bar, 60 nm. Full size image Recent studies have shown that supercrystalline SPs can be obtained through a thermal annealing process [33] , [34] , [35] . We performed a thermal annealing of our CS-SPs. TEM images show that on annealing at 80 °C for 24 h, the ‘core-shell’ structure is preserved, but the core MNPs form an ordered structure and display highly ordered and atomic-like superlattice fringes ( Fig. 2a–d ). Analyses of the observed fringes and superlattice orientations suggest that the core particles in CS-SPs form an fcc superlattice with an estimated lattice constant of 10.5±0.2 nm ( Fig. 2a–c ). 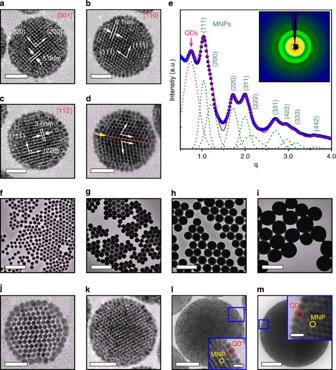Figure 2: Supercrystalline CS-SPs and their size-controlled syntheses. TEM images of supercrystalline CS-SPs viewed along different zone axes (a) [001], (b) [110] and (c). (d) TEM image of a CS-SP with a stacking fault marked with a yellow arrow. Scale bars, 50 nm (a–d). (e) The integrated data from the SAXS pattern (inset) of CS-SPs show a position ratio series ofq/q0=1////////, (q0is the position of the (111) peak,q=4πsinθ/λ), indicating an fcc close packing of the MNPs. Large-area TEM images (f–i) and higher magnification TEM images (j–m) of CS-SPs with an average diameter of 80±9 nm (f,j), 120±13 nm (g,k), 235±30 nm (h,l) and 360±60 nm (i,m). The insets inlandmare zoomed-in images of the blue squares. Scale bars, 500 nm (f–i). Scale bars, 30 nm, 50 nm, 70 nm and 100 nm (j–m), respectively. Scale bars,15 nm (insets oflandm). Red and yellow circles indicate the positons of QDs and MNPs, respectively. Figure 2a–c display typical TEM images of these crystalline CS-SPs viewed along the [001], [011] and zone axes, respectively. Typical TEM images further indicate that some CS-SPs include defects and stacking faults ( Fig. 2d ). High-resolution synchrotron small angle X-ray scattering (SAXS) characterization unambiguously confirms the assignment of a highly ordered fcc superlattice ( Fig. 2e ). The first broad SAXS peak represents strong diffuse scattering from the randomly distributed ‘shell’ QDs, but other SAXS peaks are well assigned to Bragg peaks from an ideal fcc superlattice, corresponding to the Fm3m space group ( Fig. 2e ). The calculated lattice constant is 10.4±0.2 nm ( Supplementary Table 1 ), consistent with TEM observations ( Fig. 2a–d ). Correlating the SAXS-defined nearest interparticle spacing of 7.3 nm to the average MNP size of 5.9 nm gives an interparticle distance of 1.4 nm, consistent with coiled and intercalated oleate ligands on MNPs surfaces [36] , [37] . Given the average diameter of CS-SPs, the number of MNPs inside each CS-SP is estimated at ~2,020±230, with a packing density of 39%. On fine-tuning the ratio of nanoparticles (both QDs and MNPs) to DTAB surfactant and the ratio of QDs to MNPs ( Supplementary Table 2 ), we can obtain a wide range of the crystalline CS-SPs with an average diameter ranging from ~80 to ~360 nm ( Fig. 2f–i ). Higher magnification TEM images clearly show the core-shell structure of individual crystalline SPs for all sizes ( Fig. 2j–m ). Figure 2: Supercrystalline CS-SPs and their size-controlled syntheses. TEM images of supercrystalline CS-SPs viewed along different zone axes ( a ) [001], ( b ) [110] and ( c ) . ( d ) TEM image of a CS-SP with a stacking fault marked with a yellow arrow. Scale bars, 50 nm ( a – d ). ( e ) The integrated data from the SAXS pattern (inset) of CS-SPs show a position ratio series of q/q0=1/ / / / / / / / , ( q0 is the position of the (111) peak, q = 4π sin θ/ λ), indicating an fcc close packing of the MNPs. Large-area TEM images ( f – i ) and higher magnification TEM images ( j – m ) of CS-SPs with an average diameter of 80±9 nm ( f , j ), 120±13 nm ( g , k ), 235±30 nm ( h , l ) and 360±60 nm ( i , m ). The insets in l and m are zoomed-in images of the blue squares. Scale bars, 500 nm ( f – i ). Scale bars, 30 nm, 50 nm, 70 nm and 100 nm ( j – m ), respectively. Scale bars,15 nm (insets of l and m ). Red and yellow circles indicate the positons of QDs and MNPs, respectively. Full size image With their combination of both magnetism and fluorescence, CS-SPs have potential in various applications and technological devices. However, feasible applications, especially in biological systems, often require additional surface functionality, and this can be significantly hindered with CS-SPs that have a PVP polymer surface. To overcome this challenge and improve biocompatibility and colloidal stability, we encapsulate CS-SPs (~80 nm) with a thin silica shell through a sol-gel process [38] , [39] . TEM characterization shows that each CS-SP is uniformly coated with a 10.6±0.7-nm-thick silica shell ( Fig. 3a ). Scanning TEM line scan, element mapping and three-dimensional TEM tomography show that the core-shell superstructure is preserved ( Fig. 3b , Supplementary Fig. 6 and Supplementary Movie 3 ). Dynamic light scattering measurements reveal that the HD diameter dramatically decreases from ~130 to~100 nm, similar to the TEM-determined size of ~100 nm ( Fig. 3a and Supplementary Fig. 7 ). The decrease in HD size implies a complete removal of the bulky PVP layer. Importantly, these silica-CS-SPs display a high degree of colloidal stability. No measureable changes in both the PL intensity and HD size can be observed after 6 months at 4 °C ( Fig. 3c ). These silica-CS-SPs exhibit superparamagnetism at room temperature with a saturation magnetization of 15.2 emu g −1 (1.4 × 10 −14 emu per particle) ( Fig. 3d , Supplementary Fig. 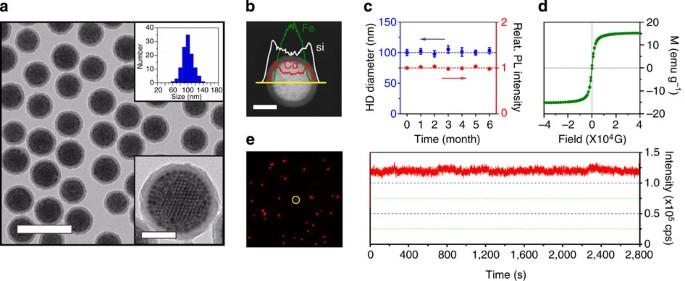Figure 3: Silica-coated CS-SPs. (a) A representative TEM image of silica-coated CS-SPs (silica-CS-SPs) with a thin layer thickness of ~10.6±0.7 nm. Scale bar, 200 nm. Insets show the histogram of the particle diameter distribution of silica-CS-SPs with an average diameter of 100±12 nm (top right) and a zoomed-in TEM image of one silica-CS-SP (bottom right). Scale bar, 50 nm (inset). (b) An image of dark-field scanning TEM and elemental line scan from a silica-CS-SP show that while maintaining the core-shell superstructure, a thin layer of silica shell is uniformly deposited onto the CS-SP’s surface. Scale bar, 50 nm. (c) HD diameter and relative photoluminescence (relat. PL) intensity of silica-CS-SPs as a function of storage time. (d) Magnetic characterization (magnetization versus magnetic field at 300 K) shows the superparamagnetism of silica-CS-SPs. (e) Left, epi fluorescence image of silica-CS-SPs on a glass substrate. Right, a representative photoluminescence time trace of a single silica-CS-SP. 8 and Supplementary Table 3 ). The decreased magnetization compared with that of free Fe 3 O 4 MNPs (63.7 emu g −1 , Supplementary Fig. 9 ) is due to non-magnetic components inside each silica-CS-SP (the QDs, the silica layer and the organic ligands) with a mass percentage of 75.2% ( Supplementary Fig. 10 and Supplementary Table 3 ). The PL QY of the silica-CS-SPs was measured to be ~12% using a 405-nm excitation light, comparable with that of the PVP-coated CS-SPs ( Supplementary Fig. 11 ). The decreased QY compared with free QDs (PL QY of 94%) is in large part a result of the MNPs strongly absorbing this wavelength light. Under the illumination of a continuous wave laser at a power density of 22 W cm −2 for ~2,800 s, silica-CS-SPs did not show evidence either of blinking or photobleaching ( Fig. 3e ), thus making them an ideal tool for single particle tracking. To demonstrate the silica-layer-enabled surface functionality, methoxy-polyethylene-glycol silane (mPEG-silane, MW 5,000gmol −1 ) was conjugated to the CS-SPs ( Supplementary Fig. 12 ). The resulting particles have nearly neutral surfaces (−5.1±2.3 mV, Supplementary Fig. 13 ), minimal cell toxicity ( Supplementary Fig. 14 ) and minimal protein adsorption ( Supplementary Fig. 15 ). These features allow for the ultimate use of these CS-SPs in various biological systems. Figure 3: Silica-coated CS-SPs. ( a ) A representative TEM image of silica-coated CS-SPs (silica-CS-SPs) with a thin layer thickness of ~10.6±0.7 nm. Scale bar, 200 nm. Insets show the histogram of the particle diameter distribution of silica-CS-SPs with an average diameter of 100±12 nm (top right) and a zoomed-in TEM image of one silica-CS-SP (bottom right). Scale bar, 50 nm (inset). ( b ) An image of dark-field scanning TEM and elemental line scan from a silica-CS-SP show that while maintaining the core-shell superstructure, a thin layer of silica shell is uniformly deposited onto the CS-SP’s surface. Scale bar, 50 nm. ( c ) HD diameter and relative photoluminescence (relat. PL) intensity of silica-CS-SPs as a function of storage time. ( d ) Magnetic characterization (magnetization versus magnetic field at 300 K) shows the superparamagnetism of silica-CS-SPs. ( e ) Left, epi fluorescence image of silica-CS-SPs on a glass substrate. Right, a representative photoluminescence time trace of a single silica-CS-SP. Full size image One of the persistent challenges in cell biology is to understand how a series of biomolecular activities can be integrated and modulated in the intracellular space. Several recent experiments have shown how MNPs could be used as actuators for remote control of signalling processes at the single cell level with subcellular resolution [40] , [41] . Yet, experimental failure is quite common, mainly due to particle polydispersities in size and magnetic content that not only make microinjection of nanoparticles difficult, but also render intracellular manipulation fragile due to the viscoelasticity of the cytoplasm. As a consequence, there is a pressing need for the fabrication of nanoparticles that have a small and uniform size but still show strong magnetism for efficient response, and are also highly fluorescent for monitoring their intracellular spatial distribution. The specifications of our silica-CS-SPs meet all these requirements. Given a particle diameter of ~100 nm, forces on the order of 1 pN, similar to the force generated by a molecular motor [42] , can be generated with a magnetic tip ( Fig. 4a ). These forces were sufficient to efficiently manipulate silica-CS-SPs across whole cells within minutes ( Fig. 4b–d and Supplementary Movies 4 and 5 ). The movement of the silica-CS-SPs appears to be only marginally hindered by the cytoplasmic meshwork ( Fig. 4b–d ). The silica-CS-SPs are bright enough that their individual trajectories can be tracked with great accuracy (a pointing accuracy of ~15 nm) throughout their transport within the cytoplasm ( Fig. 4b,c ). The key for success and reproducibility of these experiments is the superior homogeneity in both particle size and magnetic content of these silica-CS-SPs. We thus expect silica-CS-SPs, once decorated with targeting or signalling molecules, to constitute a powerful platform for the magnetic control/manipulation of intracellular processes. 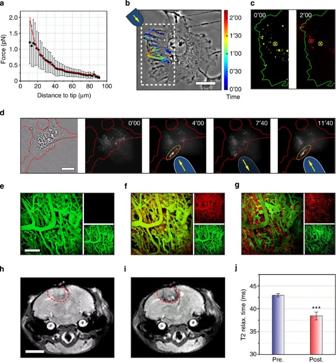Figure 4: Silica-CS-SPs in biological applications. (a) Force applied to individual silica-CS-SPs as a function of the distance from the magnetic tip (Supplementary Movie 6). A power law (red curve) fits the data. (b) Tracking of individual silica-CS-SPs during their manipulation inside a Cos7 cell (Supplementary Movie 4). Positions along each trajectory are colour-coded according to the time. Scale bar, 15 μm. (c) Left: fluorescence imaging of individual silica-CS-SPs (yellow) in the dashed line region ofband before the manipulation. The barycenter of the individual localizations is shown as a yellow cross. Right: superposition of the silica-CS-SPs fluorescence after 2 min (red), the barycenter of the individual localizations is shown as a red cross. (d) Left: transmission picture of a Hela cell in which silica-CS-SPs have been microinjected. By bringing the magnetic tip in and out (blue bars), a reversible accumulation of silica-CS-SPs (yellow region) can be created at the cell periphery (indicated by red dashed line), in the direction of the magnetic tip (Supplementary Movie 5). Scale bar, 15 μm. mPEG-silane (MW 5000) functionalized silica-CS-SPs (200 μl, 2 mg ml−1) were intravenously injected into C3H mice bearing brain metastasis of a murine mammary carcinoma (MCaIV) with a cranial window model. Intravital multiphoton microscopy through the cranial window was carried out at different time point: pre-injection (e), 4 h post injection (f) and 24 h post injection (g). Scale bar, 150 μm. Images from red and green channels are shown in small panels (top: red channel, bottom: green channel). Green emission signals are generated from a blood vessel tracer (fluorescein isothiocyanate–dextran (FITC-Dextran)) and red emission signals are generated by mPEG-functionalized silica-CS-SPs.In vivo T2-weighted magnetic resonance images of pre- (h) and 24 h post- (i) injection of mPEG-silane functionalized silica-CS-SPs. Twenty four hours post-injection image show clear tumour visualization (denoted by the red dash line). Scale bar, 3 mm. (j) The correspondingT2relaxation (relax.) time fitting results for the tumour region at time points of pre-injection (Pre., blue bar) and 24 h post injection (Post., red bar).n=5 mice, ***P<0.001 (Student’st-test). Figure 4: Silica-CS-SPs in biological applications. ( a ) Force applied to individual silica-CS-SPs as a function of the distance from the magnetic tip ( Supplementary Movie 6 ). A power law (red curve) fits the data. ( b ) Tracking of individual silica-CS-SPs during their manipulation inside a Cos7 cell ( Supplementary Movie 4 ). Positions along each trajectory are colour-coded according to the time. Scale bar, 15 μm. ( c ) Left: fluorescence imaging of individual silica-CS-SPs (yellow) in the dashed line region of b and before the manipulation. The barycenter of the individual localizations is shown as a yellow cross. Right: superposition of the silica-CS-SPs fluorescence after 2 min (red), the barycenter of the individual localizations is shown as a red cross. ( d ) Left: transmission picture of a Hela cell in which silica-CS-SPs have been microinjected. By bringing the magnetic tip in and out (blue bars), a reversible accumulation of silica-CS-SPs (yellow region) can be created at the cell periphery (indicated by red dashed line), in the direction of the magnetic tip ( Supplementary Movie 5 ). Scale bar, 15 μm. mPEG-silane (MW 5000) functionalized silica-CS-SPs (200 μl, 2 mg ml −1 ) were intravenously injected into C3H mice bearing brain metastasis of a murine mammary carcinoma (MCaIV) with a cranial window model. Intravital multiphoton microscopy through the cranial window was carried out at different time point: pre-injection ( e ), 4 h post injection ( f ) and 24 h post injection ( g ). Scale bar, 150 μm. Images from red and green channels are shown in small panels (top: red channel, bottom: green channel). Green emission signals are generated from a blood vessel tracer (fluorescein isothiocyanate–dextran (FITC-Dextran)) and red emission signals are generated by mPEG-functionalized silica-CS-SPs. In vivo T 2 -weighted magnetic resonance images of pre- ( h ) and 24 h post- ( i ) injection of mPEG-silane functionalized silica-CS-SPs. Twenty four hours post-injection image show clear tumour visualization (denoted by the red dash line). Scale bar, 3 mm. ( j ) The corresponding T 2 relaxation (relax.) time fitting results for the tumour region at time points of pre-injection (Pre., blue bar) and 24 h post injection (Post., red bar). n =5 mice, *** P <0.001 (Student’s t -test). Full size image Another biomedical application of interest of MNPs is their use as markers for MR imaging. The T 2 -weighted MR contrast is dramatically enhanced in silica-CS-SPs due to the high degree of aggregation of the core MNPs [15] , [43] , [44] , [45] , [46] , giving a T 2 relaxivity of 402.7 mM −1 S −1 , ~6.2 times larger than for the individual MNPs ( Supplementary Fig. 16 ). Such a high T 2 relaxivity coupled with excellent PL properties make silica-CS-SPs ideal MP/MR dual-modal in vivo imaging probes. As a demonstration, mPEG functionalized silica-CS-SPs with an HD diameter of ~120 nm (200 μl, 2 mg ml −1 ) were intravenously injected into mice bearing brain metastasis of a murine mammary carcinoma (MCaIV) [47] . Both the optical MP images ( Fig. 4e–g ) and T 2 -weighted MR images ( Fig. 4h–j ) reveal that silica-CS-SPs selectively accumulate in the tumour region 24 h after injection through an enhanced permeation and retention effect [48] . These experiments demonstrate the potential of our silica-CS-SPs as unique powerful in vivo MP/MR dual-modal imaging probe. In conclusion, we demonstrate a simple and effective method for assembling CdSe-CdS QDs with Fe 3 O 4 MNPs into colloidal SPs with a ‘core-shell’ superstructure. These SPs have remarkably narrow size distributions, so that the properties of single SPs reliably map onto the properties of the ensemble. Additional thermal annealing drives the crystallization of the ‘core’ MNPs into a highly ordered supercrystal with an ideal fcc superlattice. The CS-SPs can be easily coated with a thin silica layer, providing surface functionality and colloidal stability, as well as biocompatibility. Importantly, these silica-CS-SPs simultaneously exhibit uniform and tunable sizes, high magnetic content loading, maximized fluorophore loading on the surface, substantial colloidal stability and versatile surface functionality. These features allow the utilization of these magneto-fluorescent SPs for in vitro intracellular manipulation and in vivo MR/MP dual-mode imaging. Given the versatility of our assembly strategy, we anticipate that driven by various applications, SPs with a variety of compositions will also be achieved using this method. Synthesis of QDs and MNPs nanocrystals High-quality uniform CdSe-CdS core-shell QDs and Fe 3 O 4 MNPs with tunable sizes are synthesized according to the literature methods [49] , [50] . Detailed information regarding synthesis can be found in the Supplementary Methods . As-synthesized nanocrystals were purified by precipitation with acetone and were dispersed in chloroform to form stock solutions with concentrations of 20–50 mg ml −1 . Synthesis of CS-SPs with a random magnetic ‘core’ In a typical synthesis, 1 ml chloroform solution containing 4 mg 9.0-nm QDs and 6 mg 5.9-nm MNPs was injected to 1 ml DTAB aqueous solution (20 mg ml −1 in Nanopure water). The solution was thoroughly mixed by vortex for 5 s. After removing the chloroform from the mixture by blowing Ar at room temperature, a clear QD-MNP-micelle aqueous solution was obtained. This QD-MNP-micelle solution was swiftly injected into a 5-ml PVP (MW 55,000) EG solution (2 mM) under vigorous stirring with a stirring speed of 700 r.p.m. for 30 min at room temperature. The resulting CS-SPs were isolated by centrifugation, re-dispersed in ethanol and stored at ~4 °C. Synthesis of CS-SPs with a supercrystalline magnetic core The synthesis procedure is the same as the synthesis of CS-SPs described above, except that an additional thermal annealing process was carried out after the CS-SPs synthesis. In this thermal annealing process, the resulting CS-SPs in PVP/EG solution was heated to 80 °C with a slow stirring speed (300 r.p.m.) and kept for 24 h before cooling to room temperature. The resulting supercrystalline CS-SPs were isolated by centrifugation, redispersed in ethanol and stored at ~4 °C as a stock solution. Synthesis of silica-CS-SPs For a typical synthesis, 2 mg CS-SPs was dissolved in 20 ml ethanol. Under vigorous stirring, 3 ml deionized water (DI water) and 1 ml NH 3 ·H 2 O solution was added dropwise in the reaction solution, followed by the addition of 50 μl TEOS. The final solution was kept stirring at room temperature for 20 min. The resulting silica-CS-SPs were isolated by centrifugation, washed with DI water, dissolved in 2 ml DI water and stored at ~4 °C. Synthesis of mPEG-silane functionalized silica-CS-SPs Two millilitres of silica-CS-SPs were diluted in 10 ml DI water. Under magnetic stirring, 50 μl NH 3 ·H 2 O solution and 20 μl TEOS were added into the solution, sequentially. After the mixture solution was heated to 70 °C, 1 ml mPEG-silane (MW 5,000) aqueous solution (0.02 M) was dropped in. The reaction solution was kept stirring at 70 °C for 3 h and then stirred at room temperature for another 15 h. The resulting mPEG-silane functionalized silica-CS-SPs were isolated by centrifugation, washed three times with nanopure water and finally dissolved in 1 ml phosphate buffer solution (PBS, 1 × ) and stored at ~4 °C fridge. Magnetic manipulation of the silica-CS-SPs in living cells For manipulation in living cells, HeLa cells and Cos7 cell lines were cultured at 37 °C in 5% CO 2 in DMEM supplemented with 10% FCS. For imaging and manipulation, cells were grown on 25 mm glass coverslips. Experiments were performed at 37 °C in a heating chamber placed on the inverted microscope. Microinjection was performed with the same borosilicate needles as described above and filled with a concentrated solution of SPs. After microinjection, the cells were left for 20 min recovery. To bring the tip close to the sample with the orientation adapted to each unique cell morphology, the magnetic tip was attached to a circular teflon holder, allowing us to rotate the tip in respect to the optical axis of the microscope, as described in Etoc et al . [41] Tracking of the manipulated SPs was performed semi-manually using the Manual Tracking plugin of ImageJ. Intravital multiphoton microscopy All animal procedures were carried out following the Public Health Service Policy on Humane Care of Laboratory Animals and approved by the Institutional Animal Care and Use Committee of the Massachusetts General Hospital. Imaging studies were carried out using an MCaIV cranial window model in C3H mice [51] . MCaIV tumour cell pellet (~2.5 × 10 5 cells) is injected into the exposed parenchymal space at about 0.1 mm depth. In vivo imaging is performed on established tumours on day 9 after pellet implantation. In vivo imaging: Fluorescein isothiocyanate–dextran/PBS solution was prepared for in vivo vessel tracing in a concentration of 10 mg ml −1 . Following tail vain injection of 100 μl of fluorescein isothiocyanate–dextran, a baseline vessel image was acquired using multiphoton imaging described previously [47] on a custom-built multiphoton laser-scanning microscope using confocal laser-scanning microscope body (Olympus 300, Optical Analysis Corp.) and a broadband femtosecond laser source (High Performance MaiTai, Spectra-Physics). After acquisition of a baseline image, mPEG-silane functionalized silica-CS-SPs solution (200 μl, 2 mg ml −1 ) were intravenously injected via tail vein. Image slices were taken with 400 mW at a wavelength of 820 nm in three ROIs in tumour area and one in the healthy contralateral hemisphere. Images were taken with depths from 0 to 150 μm. Imaging studies were performed with a × 20 magnification, 0.95 numerical aperture water-immersion objective (Olympus XLUMPlanFl, 1-UB965, Optical Analysis). Image analysis was carried out using ImageJ. In vivo magnetic resonance imaging study All experiments were performed on a 9.4 T magnet (Magnex Scientific Ltd, Oxford, UK) equipped with a 60-mm inner diameter gradient coil (Resonance Research, Billerica, MA) and interfaced with a Bruker MRI console (Bruker Biospin, Billerica, MA). The gradient coil has a maximum strength of 1,500 mT m −1 and a rise time of 100 μs. Images were acquired using a home-built mouse head bird-cage coil. Mice were positioned on a custom-made mouse cradle and anaesthetized with 1.5% isoflurane in 50/50 O 2 /medical air mixture with total flow rate of 1,200 ml min −1 . T 2 -weighted RARE MRI: . T 2 -weighted rapid acquisition with refocused echoes (RARE) images were acquired with the following acquisition parameters: echo time (TE)=10, RARE factor=8, repetition time (TR)=2,500 ms, numerical aperture=4, 15 image slices, 0.5 mm slice thickness, 125 μm in-plane resolution. Tumour volume was determined from the T 2 hyperintense tumour region of the brain. T 2 maps: . T 2 maps were generated from multi-echo spin-echo and multi-echo gradient-echo images, respectively, using a custom-written MATLAB programme for voxel-wise fitting of the T 2 relaxation times. Multi-echo spin-echo image acquisition parameters were: TE=10 ms, 15 echoes with 10 ms increment, TR=2.5 s, 2 averages, field of view (FOV)=1.6 cm, matrix=128 × 128 (in-plane resolution 125 μm), slice thickness=0.5 mm and 15 image slices. Multi-echo gradient-echo image acquisition parameters were: TE=2.5 ms, 10 echoes with 2.5 ms increment, TR=1.5 s, 4 averages, FOV=1.6 cm, matrix=96 × 96, slice thickness=0.5 mm and 15 image slices. How to cite this article: Chen, O. et al . Magneto-fluorescent core-shell supernanoparticles. Nat. Commun. 5:5093 doi: 10.1038/ncomms6093 (2014).